Translation of HTT mRNA with expanded CAG repeats is regulated by the MID1–PP2A protein complex Expansion of CAG repeats is a common feature of various neurodegenerative disorders, including Huntington’s disease. Here we show that expanded CAG repeats bind to a translation regulatory protein complex containing MID1, protein phosphatase 2A and 40S ribosomal S6 kinase. Binding of the MID1–protein phosphatase 2A protein complex increases with CAG repeat size and stimulates translation of the CAG repeat expansion containing messenger RNA in a MID1-, protein phosphatase 2A- and mammalian target of rapamycin-dependent manner. Our data indicate that pathological CAG repeat expansions upregulate protein translation leading to an overproduction of aberrant protein and suggest that the MID1-complex may serve as a therapeutic target for the treatment of CAG repeat expansion disorders. Huntington’s disease (HD) (OMIM accession code 143100) is caused by an expanded CAG repeat in exon 1 of the Huntingtin (HTT ) gene. HD is characterized by progressive neuronal cell death associated with choreatic movements, as well as dementia. The disease progresses over time and is invariably fatal. In most cases onset occurs in mid-life (35–50 years). Age at onset is inversely correlated to the length of the extensions of the CAG stretches (reviewed in Gil and Rego [1] ). A pathological hallmark of several CAG repeat expansion disorders is the formation of protein aggregates in neurons. Expanded CAG sequences are translated into elongated polyglutamine (polyQ) stretches. This renders the respective proteins insoluble and leads to the formation of protein aggregates [2] , [3] , [4] , [5] , [6] , [7] . In some CAG repeat expansion disorders gain-of-function at the RNA instead of the protein level has been proposed [8] . CAG sequences form double-stranded RNA structures, the stability of which increases with repeat-numbers [9] , [10] , [11] . For example the CAG repeat region of the HTT messenger RNA (mRNA) forms double-stranded hairpin structures [12] . Some proteins bind to such CAG structures in a repeat size-dependent manner [13] . Thus, it is thought that expansion of CAG repeat structures leads to the formation of pathological RNA–protein complexes, which cause damage in both—the nucleus where they influence the splicing machinery–and in the cytosol where they interfere with mRNA processing and translation [12] , [14] . Several processes in gene expression, from mRNA transcription and stability to translation, involve RNA-binding proteins, which assemble with the mRNAs into mRNP (messenger ribonucleoprotein) complexes [15] . One of such mRNP complexes contains the MID1 protein, the catalytic subunit of protein phosphatase 2A (PP2Ac) and 40S ribosomal S6 kinase (S6K), a target of mammalian target of rapamycin (mTOR) kinase and PP2A [16] , [17] . MID1 is a ubiquitin ligase that binds the α4 protein, a regulatory subunit of PP2A. Through this interaction MID1 ubiquitinates PP2Ac and targets it towards ubiquitin-specific degradation by the proteasome. Therefore, MID1 is a negative regulator of PP2Ac [18] . Through this negative regulatory influence on PP2A activity, MID1 also controls the activity of the mTOR kinase. High levels of PP2A activity in MID1-deficient cells abolish the interaction between mTOR and raptor, which is an essential cofactor of mTOR activity [19] . Accordingly, a significant reduction of mTOR activity is found in these cells. mTOR and its counteracting phosphatase PP2A have important roles in the regulation of protein translation. Both enzymes control the phosphorylation and thereby the activity of several translation regulators. For example, mTOR phosphorylates and activates S6K and 4E-BP1, both of which participate in the assembly of the eukaryotic translation initiation factor (elF)3 complex and the initiation of translation: when inactive, S6K associates with the elF3 preinitiation complex. Upon stimulation mTOR localizes to the elF3 complex and activates S6K via phosphorylation [20] , [21] . Activated S6K phosphorylates and enhances the activity of its targets elF4B and S6 (ref. 21 ). The 5′-untranslated region (UTR) of specific mRNAs folds into stable secondary structures, which principally suppress protein translation [22] , [23] . Activated elF4B unwinds and linearizes such UTRs, allowing initial binding of the 40S ribosome and scanning towards the translation initiation codon [24] , [25] . Concurrently mTOR phosphorylates 4E-BP1, an inhibitory regulator of elF4E, leading to dissociation of 4E-BP1 from the cap complex, thereby allowing binding of elF4E to elF4G and assembly of the preinitiation complex finally resulting in translation initiation [21] , [25] . mTOR dependent phosphorylation of S6K and 4E-BP1, therefore, efficiently supports protein translation, while their dephosphorylation by PP2A inhibits it. Besides regulating PP2A and mTOR activities, the MID1-complex contains polyribosomes and several translation factors and is able to bind mRNA thereby forming a microtubule-associated mRNP complex [17] . As we have shown previously MID1 and α4 stimulate translation of mRNAs that are associated with the MID1 protein complex [16] . Here we demonstrate that the MID1 protein together with its interaction partners PP2A and S6K binds mutant HTT mRNA via its elongated CAG repeats. This interaction results in enhanced translation of mutant HTT mRNA, an effect that can be significantly reduced by knockdown of MID1. The PP2A inhibitor okadaic acid (OA) can block this reduction in translation caused by MID1 knockdown. Furthermore, the mTOR inhibitor temsirolimus can block the increased translation of HTT mRNA with expanded CAG repeats. Taken together our data indicate that expanded CAG repeats in mRNAs trigger translation in a MID1/PP2A/mTOR dependent manner and they suggest that the MID1-complex might be a novel, promising drug target for the development of therapeutic strategies against CAG repeat expansion disorders like HD. MID1-complex binds CAG repeats in a length dependent manner CAG repeat RNAs fold into secondary hairpin structures [9] , [10] , [11] , [12] . To give an idea of how these hairpins could look like, we performed in silico RNA-structure predictions of CAG repeat stretches with different repeat sizes. A CAG-containing loop that elongates with increasing CAG number is particularly pronounced ( Supplementary Fig. S1 ). The MID1 protein complex binds mRNAs through G-rich RNA motifs forming stable secondary structures [16] , [17] , [26] . Thus, CAG repeat stretches, which are G-rich structures and form stable hairpins, could be recognized by the MID1-complex. To test this, we performed RNA–protein pull-down assays. Equal amounts of in vitro transcribed, biotinylated HTT-exon1-mRNA carrying either 20 (representing physiological numbers of repeats) or 51 (representing pathological numbers of repeats) CAG repeats were incubated with HeLa cell extracts that either contained FLAG-MID1 ( Fig. 1a ) or no recombinant protein ( Fig. 1b ). RNAs were purified with streptavidin-coated beads and bound proteins were analysed by western blotting using (i) an anti-FLAG antibody ( Fig. 1a ), (ii) an antibody detecting endogenous MID1 ( Fig. 1b ) and (iii) an antibody detecting glyceraldehyde 3-phosphate dehydrogenase as a negative control that does not bind to the MID1 protein complex. In addition, an experiment without RNA was performed. Although binding of MID1 to the 20 CAG, repeat RNA was weak, a strong band of the MID1 protein (FLAG-tagged and endogenous) was detected in the sample with the 51 repeat RNA. Glyceraldehyde 3-phosphate dehydrogenase did not bind to any of the RNAs. 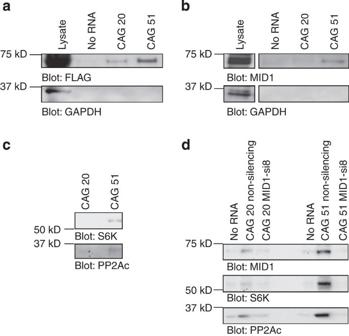Figure 1: The MID1-complex binds CAG-repeat-motifs in a size-dependent manner. (a) RNA–protein pull-down of FLAG-MID1 with RNA containing 20 or 51 CAG repeats (CAG 20, CAG 51) or without RNA (no RNA). RNA-bound proteins were analysed on western blots detecting FLAG-MID1. Glyceraldehyde 3-phosphate dehydrogenase (GAPDH) was detected as negative control that does not bind to the MID1 protein complex. (b) RNA–protein pull-down of endogenous MID1 as in (a). (c) RNA–protein pull-down assay as described in (a). RNA-bound proteins were analysed on a western blot using specific antibodies detecting PP2Ac and S6K. (d) RNAse assisted chromatography of protein lysates from cells transfected with non-silencing control or MID1-specific siRNAs. Proteins bound to RNA containing 20 or 51 CAG repeats were analysed on a western blot using specific antibodies detecting MID1, PP2Ac and S6K. An experiment without RNA (no RNA) was included as negative control. Figure 1: The MID1-complex binds CAG-repeat-motifs in a size-dependent manner. ( a ) RNA–protein pull-down of FLAG-MID1 with RNA containing 20 or 51 CAG repeats (CAG 20, CAG 51) or without RNA (no RNA). RNA-bound proteins were analysed on western blots detecting FLAG-MID1. Glyceraldehyde 3-phosphate dehydrogenase (GAPDH) was detected as negative control that does not bind to the MID1 protein complex. ( b ) RNA–protein pull-down of endogenous MID1 as in ( a ). ( c ) RNA–protein pull-down assay as described in ( a ). RNA-bound proteins were analysed on a western blot using specific antibodies detecting PP2Ac and S6K. ( d ) RNAse assisted chromatography of protein lysates from cells transfected with non-silencing control or MID1-specific siRNAs. Proteins bound to RNA containing 20 or 51 CAG repeats were analysed on a western blot using specific antibodies detecting MID1, PP2Ac and S6K. An experiment without RNA (no RNA) was included as negative control. Full size image Furthermore, the MID1 interacting proteins of the PP2A/mTOR signalling cascade, PP2Ac and S6K, also bound to RNA containing 51 CAG repeats, while no or only very weak binding was observed with RNA containing 20 CAG repeats ( Fig. 1c ). MID1 dependency of the binding of S6K and PP2Ac to HTT mRNAs with expanded CAG repeats was tested in an RNAse assisted chromatography [27] in cells with and without MID1 knockdown. Equal amounts of in vitro transcribed HTT-exon1-mRNA with either 20 or 51 CAG repeats were incubated with cell lysates that were either transfected with non-silencing control or MID1-specific short interfering RNA (siRNA) oligonucleotides. RNAs were immobilized on magnetic beads and RNA-bound proteins were eluted from the beads using RNAse. RNA-bound proteins were analysed by western blotting using antibodies detecting MID1, S6K and PP2Ac. As a negative control an experiment without RNA was performed. Although binding of MID1, S6K, and PP2Ac to the 20 CAG repeat RNA was weak, strong bands of the three proteins were detected in the sample with the 51 repeat RNA. In the MID1 knockdown samples neither MID1 nor S6K or PP2Ac could be detected in the elution fraction suggesting that MID1 mediates binding of S6K and PP2Ac to the CAG repeat containing RNA ( Fig. 1d , for knockdown control see Supplementary Fig. S2 ). The preceding data suggest that longer CAG repeats bind the MID1 protein complex more efficiently than shorter. In order to verify this, we repeated the RNA–protein pull-down experiment using HeLa cells overexpressing MID1-FLAG with increasing salt concentrations. At 100 mM salt both RNAs, with 20 and 51 CAG repeats bound MID1 and PP2Ac. At 150 and 200 mM the 20 CAG repeat containing RNA lost MID1 and PP2Ac-binding capabilities. By contrast, significant amounts of MID1 and PP2Ac were still bound to the CAG 51 containing RNA ( Supplementary Fig. S3 ) suggesting that the binding affinity of the MID1 protein complex increases with the length of the repeat. HTT translation increases with the number of CAG repeats The experiments described above, and the role of the MID1 protein complex in the regulation of translation efficiency of mRNAs specifically attached to it [16] made us hypothesize that (i) the MID1-complex could control the translation of mRNAs with expanded CAG repeats, and (ii) the amount of protein that is synthesized from a CAG repeat containing mRNA increases with the length of the repeat. To examine whether the repeat size influences the amount of translated protein, mouse embryonic fibroblasts (Atg +/+) were transfected with expression-vectors producing an N-terminal HTT-fragment covering the first 500 amino acids (HTT-500AA) with either 17 or 49 glutamines (Q) together with a green fluorescent protein (GFP)-expression vector as an internal transfection control. Cell extracts were analysed by western blotting. For quantification HTT-500AA signals were related to GFP and Q17 expression was set to 1. A significantly higher production of protein with 49 than with 17 Q-repeats was revealed ( Fig. 2a ). 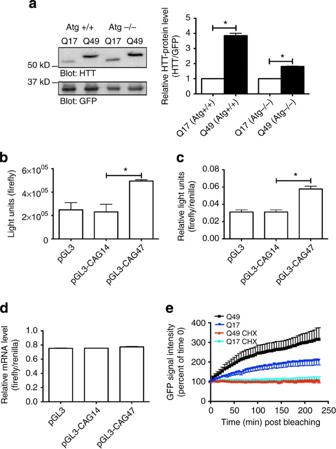Figure 2: Protein synthesis increases with repeat sizein vitro. (a) Expression of the first 500 amino acids of the human Huntingtin protein carrying either 17 (HTT-500AA-Q17) or 49 glutamines (HTT-500AA-Q49) in autophagy positive (Atg +/+) and autophagy negative (Atg −/−) cells is shown. Left: western blot analysis of Atg +/+ and Atg −/− cells co-transfected with pEGFP-C1 and HTT-500AA-Q17/HTT-500AA-Q49. Right: quantifications of relative HTT-500AA protein normalized to GFP are shown, signals for Q17 were set to 1. Samples were measured in triplicates. Mean values±s.d. are shown.P<0.001. (b)In vitrotranslation assay of firefly luciferase carrying no, 14, or 47 CAG repeats in its 3′-UTR (pGL3, pGL3-CAG14, pGL3-CAG47). Firefly activity is shown. Samples were measured in triplicates. Mean values±s.d. are shown.P<0.000002. (c) Dual-luciferase assay of U373MG-cells transfected with constructs used inbis shown. Columns represent light units of firefly luciferase normalized to renilla. Samples were measured in triplicates. Mean values±s.d. are shown.P<0.0004. (d) Real-time PCR analysis of cells fromcmeasuring firefly luciferase-mRNA expression normalized to renilla mRNA expression is shown. Samples were measured in quadruplicates. Mean values±s.d. are shown. (e) FRAP-based assay showing GFP-HTT-exon1 translation in living cells. HeLa cells were transfected with GFP-HTT-exon1 constructs, either containing 17 CAG (Q17,n=32) or 49 CAG repeats (Q49,n=16). Twelve hours after transfection cells were bleached and recovery of green fluorescence was measured. Also, analysis of the GFP-HTT-exon1 Q17 (n=28) and Q49 (n=27) constructs with cycloheximide (CHX) is shown. GFP-signal recovery over time is shown. Lines represent mean values of all cells analysed. Data are presented as mean values±s.e.m. Q17 versus Q49P<0.0001, Q49 versus Q49+CHXP<0.0001. Figure 2: Protein synthesis increases with repeat size in vitro. ( a ) Expression of the first 500 amino acids of the human Huntingtin protein carrying either 17 (HTT-500AA-Q17) or 49 glutamines (HTT-500AA-Q49) in autophagy positive (Atg +/+) and autophagy negative (Atg −/−) cells is shown. Left: western blot analysis of Atg +/+ and Atg −/− cells co-transfected with pEGFP-C1 and HTT-500AA-Q17/HTT-500AA-Q49. Right: quantifications of relative HTT-500AA protein normalized to GFP are shown, signals for Q17 were set to 1. Samples were measured in triplicates. Mean values±s.d. are shown. P <0.001. ( b ) In vitro translation assay of firefly luciferase carrying no, 14, or 47 CAG repeats in its 3′-UTR (pGL3, pGL3-CAG14, pGL3-CAG47). Firefly activity is shown. Samples were measured in triplicates. Mean values±s.d. are shown. P <0.000002. ( c ) Dual-luciferase assay of U373MG-cells transfected with constructs used in b is shown. Columns represent light units of firefly luciferase normalized to renilla. Samples were measured in triplicates. Mean values±s.d. are shown. P <0.0004. ( d ) Real-time PCR analysis of cells from c measuring firefly luciferase-mRNA expression normalized to renilla mRNA expression is shown. Samples were measured in quadruplicates. Mean values±s.d. are shown. ( e ) FRAP-based assay showing GFP-HTT-exon1 translation in living cells. HeLa cells were transfected with GFP-HTT-exon1 constructs, either containing 17 CAG (Q17, n =32) or 49 CAG repeats (Q49, n =16). Twelve hours after transfection cells were bleached and recovery of green fluorescence was measured. Also, analysis of the GFP-HTT-exon1 Q17 ( n =28) and Q49 ( n =27) constructs with cycloheximide (CHX) is shown. GFP-signal recovery over time is shown. Lines represent mean values of all cells analysed. Data are presented as mean values±s.e.m. Q17 versus Q49 P <0.0001, Q49 versus Q49+CHX P <0.0001. Full size image Autophagy has previously been shown to have an important role in the clearance of protein with polyQ stretches [28] . To exclude that unbalanced autophageal degradation causes the seen effect, the above-mentioned experiments were repeated in autophagy negative mouse embryonic fibroblasts, which were derived from mice deficient for Atg5 (Atg −/−) [29] . While expression of the HTT-500AA-Q49 protein was still significantly higher than of the Q17 protein, the difference between the Q49 and the Q17 protein was smaller in the Atg −/− cells than in the Atg +/+ cells ( Fig. 2a ). The observed differences in protein expression between both cell lines could be partially caused by autophageal imbalances that favour protein with shorter Q-stretches. The difference seen between the Q49 and Q17 in the Atg −/−, however, is caused by an autophagy independent mechanism. No differences in levels of the mRNAs of the Q49 and Q17 constructs were detected in both cell lines ( Supplementary Fig. S4 ) suggesting that differences in the translation efficiency underlie the seen effects ( Fig. 2a ). In a complementary set of experiments, low and high-number CAG repeats were cloned into the 3′-UTR of a gene encoding firefly luciferase. These reporter constructs permitted the analysis of effects mediated by CAG repeats in the mRNA without being translated into polyQ stretches. Three different constructs (empty vector: pGL3, pGL3-CAG14 and pGL3-CAG47) were subjected to an in vitro translation assay, where equal amounts of in vitro transcribed RNA from the luciferase constructs were in vitro translated in rabbit reticulocyte extracts (schematic of assay details see Supplementary Fig. S5 ). No difference in luciferase activities between the empty vector and the construct carrying 14 CAG repeats, but a significant increase in firefly activity in the sample with 47 CAG repeats was observed ( Fig. 2b ), indicating that the mRNA with a pathogenic CAG repeat is translated more efficiently than the mRNA with a non-pathogenic CAG sequence. This finding could be confirmed in U373MG-cells, a glial cell line isolated from an astrocytoma, which were transfected with the previously described luciferase constructs using a dual-luciferase reporter assay. This system is based on the co-transfection of a firefly luciferase construct with a renilla luciferase construct to control for transfection efficiency. Although there was no significant difference between the empty vector and the construct carrying 14 CAG repeats, a clear increase in firefly luciferase activity was seen with the 47 CAG repeat construct ( Fig. 2c ). By contrast, no difference between the different constructs on the mRNA level was observed ( Fig. 2d ). This provides evidence that increased firefly luciferase activity of the 47 CAG repeat construct was due to increased translation. Similar results were obtained in HeLa cells ( Supplementary Fig. S6a,b ). While also coding for glutamine on the protein levels, CAA codons do not form hairpin structures and have been shown to interrupt secondary structures formed by CAG repeats [9] , [30] . In order to test if the hairpin structure is necessary for the seen effect on luciferase activity, luciferase reporter assays using constructs in which the CAG repeats are interrupted by CAA triplets (for exact sequence see Supplementary Table S1 , structural predictions see Supplementary Fig. S7a ) have been performed. Clearly, insertion of CAA interruptions into the CAG repeat led to a significant reduction in luciferase signal ( Supplementary Fig. S7b ). Additionally, we developed a novel live-cell imaging assay based on FRAP (fluorescence recovery after photobleaching) to monitor translation. In contrast to standard FRAP applications, which are used to monitor diffusion/transport of fluorescently labelled proteins after bleaching of a defined area in the cell, we used FRAP in a whole-cell experimental set-up. Reporter constructs carrying HTT exon1 with 17 or 49 CAGs fused to GFP were transfected into HeLa cells. Twelve hours after transfection the entire cell was bleached and recovery of the fluorescent signal was monitored over 4 h. By bleaching the entire cell, we prohibited signal recovery due to diffusion of fluorescently labelled proteins into the imaging area. Therefore, only newly synthesized GFP-protein could be imaged. Clearly, GFP synthesized from a Q49 construct recovered significantly faster than from the Q17 construct ( Fig. 2e , Supplementary Movie 1 and 2 , Supplementary Fig. S8 ). Neither differences on the mRNA levels ( Supplementary Fig. S9a ) nor different transfection efficiencies of the two constructs were observed ( Supplementary Fig. S9b ). To further verify, that the fluorescence recovery was caused by newly synthesized protein, we performed the same experiment with the translation inhibitor cycloheximide. As shown in Fig. 2e (and Supplementary Movie 3 ), cycloheximide completely blocked the GFP-signal recovery. To analyse if an expanded CAG repeat stretch leads to an increase in protein production also in vivo , a knock-in mouse model for HD (B6.129-Htt tm5Mem /J, Jackson’s Lab stock no.003598), which carries 111 CAG repeats in exon 1 of the endogenous murine HTT -gene was used. Brain lysates from 2-months-old mice (wild-type, heterozygous and homozygous mutation carrier) were analysed on western blots using an HTT-antibody detecting the region N-terminal of the CAG repeat. A smaller band corresponding to wild-type HTT protein and a bigger band corresponding to mutant HTT protein, were detected. Significantly more mutant than wild-type protein was detected suggesting that the translation rate of RNA from the mutated allele is higher than from the wild-type allele in heterozygous and homozygous animals ( Fig. 3a ). Together with previous reports showing that mRNA levels of mutant HTT decrease with increasing repeat lengths in HD mouse models [31] , [32] , these data support the hypothesis that an expanded CAG repeat increases the translation efficiency of mutant HTT mRNA in vivo . 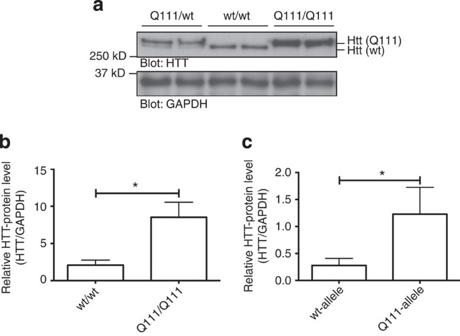Figure 3: Protein level increases with repeat sizein vivo. (a) Western blot analysis of brain extracts from wild-type (wt), heterozygous (Q111/wt) and homozygous (Q111/Q111) knock-in mice carrying 111 CAG repeats in exon 1 of HTT is shown. Two HTT bands were detected, one smaller translated from the wild-type, one bigger translated from the mutant allele. Glyceraldehyde 3-phosphate dehydrogenase (GAPDH) was analysed as control. (b) Quantifications of bands from homozygous and wild-type animals fromaare shown. (c) Quantifications of bands from heterozygous animals (protein expressed from the wild-type compared with protein expressed from the mutant allele) fromaare shown. Three animals of each genotype were quantified. Mean values±s.d. are shown.P<0.007. Figure 3: Protein level increases with repeat size in vivo . ( a ) Western blot analysis of brain extracts from wild-type (wt), heterozygous (Q111/wt) and homozygous (Q111/Q111) knock-in mice carrying 111 CAG repeats in exon 1 of HTT is shown. Two HTT bands were detected, one smaller translated from the wild-type, one bigger translated from the mutant allele. Glyceraldehyde 3-phosphate dehydrogenase (GAPDH) was analysed as control. ( b ) Quantifications of bands from homozygous and wild-type animals from a are shown. ( c ) Quantifications of bands from heterozygous animals (protein expressed from the wild-type compared with protein expressed from the mutant allele) from a are shown. Three animals of each genotype were quantified. Mean values±s.d. are shown. P <0.007. Full size image MID1 regulates translation of CAG repeat mRNAs To assess the importance of the MID1 protein for CAG repeat dependent translation, we performed MID1 knockdown before the dual-luciferase reporter assay. While mRNA levels were unaffected by the knockdown of MID1 ( Fig. 4a , for knockdown control see Fig.4c ), MID1 knockdown led to a significant reduction of the reporter signal produced by the CAG47-repeat-construct ( Fig. 4b ). By contrast, neither the luciferase signal of the empty vector control nor of the construct with 14 CAGs were affected by the MID1 knockdown, suggesting a gain-of-function of the MID1-complex on mRNAs with pathologically expanded CAG repeat stretches. Alternative MID1-targeting siRNA oligonucleotides were used to confirm these findings ( Supplementary Fig. S10 ). 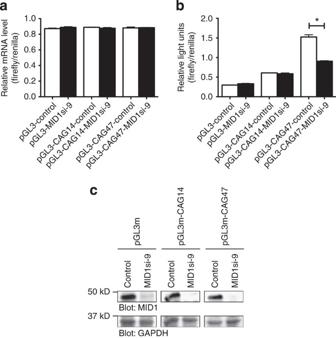Figure 4: The MID1-complex regulates translation of mRNAs with expanded CAG repeats. Dual-luciferase assays of HeLa cells are shown expressing the firefly luciferase constructs fromFig. 2co-transfected with either non-silencing (pGL3-control, pGL3-CAG14-control, pGL3-CAG47-control) or MID1-specific siRNA oligonucleotides (pGL3-MID1si-9, pGL3-CAG14-MID1si-9, pGL3-CAG47-MID1si-9). (a) Real-time PCR analysis showing relative of firefly to renilla mRNA expression. Samples were measured in quadruplicates. (b) Cells fromawere analysed for luciferase activity. Columns represent relative light units (firefly/renilla). Samples were measured in triplicates. Mean values±s.d. are shown.P<0.001. (c) Western blots for knockdown control of cells fromadetected with MID1-specific and glyceraldehyde 3-phosphate dehydrogenase (GAPDH)-specific antibodies are shown. Figure 4: The MID1-complex regulates translation of mRNAs with expanded CAG repeats. Dual-luciferase assays of HeLa cells are shown expressing the firefly luciferase constructs from Fig. 2 co-transfected with either non-silencing (pGL3-control, pGL3-CAG14-control, pGL3-CAG47-control) or MID1-specific siRNA oligonucleotides (pGL3-MID1si-9, pGL3-CAG14-MID1si-9, pGL3-CAG47-MID1si-9). ( a ) Real-time PCR analysis showing relative of firefly to renilla mRNA expression. Samples were measured in quadruplicates. ( b ) Cells from a were analysed for luciferase activity. Columns represent relative light units (firefly/renilla). Samples were measured in triplicates. Mean values±s.d. are shown. P <0.001. ( c ) Western blots for knockdown control of cells from a detected with MID1-specific and glyceraldehyde 3-phosphate dehydrogenase (GAPDH)-specific antibodies are shown. Full size image Furthermore, we utilized a cell culture model for HD. HEKT-cell lines stably expressing HTT-exon 1 with either 20, 51 or 83 CAG repeats were transfected either with MID1- or non-silencing control siRNA oligonucleotides. Cells were analysed for HTT-exon 1 protein expression either by western blotting or, for aggregate formation, in a filter-aggregation assay, which was developed by Wanker et al [33] . While the knockdown of MID1 (knockdown control see Supplementary Fig. S11 ) did not influence the synthesis of HTT-exon 1 Q20 protein ( Fig. 5a ), the expression of HTT-exon 1 Q51 ( Fig. 5b ) and the formation of aggregates by HTT-exon 1 Q83 protein ( Fig. 5c ) decreased significantly after knockdown of MID1. RNA levels were not affected by MID1 knockdown ( Fig. 5d ). 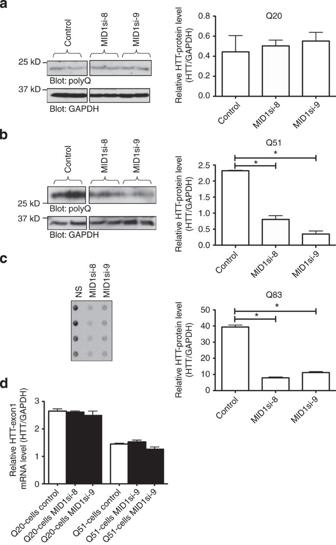Figure 5: MID1 regulates expression of aberrant HTT protein in a tissue culture model of HD. (a) Western blot analysis of cells stably expressing HTT-exon1 with 20 CAG repeats (Q20) after transfection with either non-silencing control or MID1-specific siRNA oligonucleotides (MID1si-8, MID1si-9). Western blots showing HTT-exon1 (left), and quantifications of the bands (right) are shown. Samples were measured in triplicates. Mean values±s.d. are shown.P<0.004. (b) Western blot analysis of cells stably expressing HTT-exon1 with 51 CAG repeats (Q51) after transfection with either non-silencing control or MID1-specific siRNA oligonucleotides (MID1si-8, MID1si-9). Western blots showing HTT-exon1 (left), and quantifications of the bands (right) are shown. Samples were measured in triplicates. Mean values±s.d. are shown.P<0.004. (c) Filter-aggregation assay of HEKT-cells stably expressing HTT-exon1 with 83 CAG repeats (Q83) after transfection with either non-silencing control or MID1-specific siRNA oligonucleotides (MID1si-8, MID1si-9) is shown. HTT-aggregate detection (left), and quantifications (right) are shown. Samples were measured in triplicates. Mean values±s.d. are shown.P<0.00002. (d) Real-time PCR analysis of samples fromaandbanalysing HTT-exon1-mRNA expression normalized to glyceraldehyde 3-phosphate dehydrogenase (GAPDH). Samples were measured in quadruplicates. Mean values±s.d. are shown. Figure 5: MID1 regulates expression of aberrant HTT protein in a tissue culture model of HD. ( a ) Western blot analysis of cells stably expressing HTT-exon1 with 20 CAG repeats (Q20) after transfection with either non-silencing control or MID1-specific siRNA oligonucleotides (MID1si-8, MID1si-9). Western blots showing HTT-exon1 (left), and quantifications of the bands (right) are shown. Samples were measured in triplicates. Mean values±s.d. are shown. P <0.004. ( b ) Western blot analysis of cells stably expressing HTT-exon1 with 51 CAG repeats (Q51) after transfection with either non-silencing control or MID1-specific siRNA oligonucleotides (MID1si-8, MID1si-9). Western blots showing HTT-exon1 (left), and quantifications of the bands (right) are shown. Samples were measured in triplicates. Mean values±s.d. are shown. P <0.004. ( c ) Filter-aggregation assay of HEKT-cells stably expressing HTT-exon1 with 83 CAG repeats (Q83) after transfection with either non-silencing control or MID1-specific siRNA oligonucleotides (MID1si-8, MID1si-9) is shown. HTT-aggregate detection (left), and quantifications (right) are shown. Samples were measured in triplicates. Mean values±s.d. are shown. P <0.00002. ( d ) Real-time PCR analysis of samples from a and b analysing HTT-exon1-mRNA expression normalized to glyceraldehyde 3-phosphate dehydrogenase (GAPDH). Samples were measured in quadruplicates. Mean values±s.d. are shown. Full size image Translation of CAG repeat mRNAs is PP2A and mTOR dependent MID1 is closely connected with PP2A and mTOR. In order to further confirm the interaction of MID1 and α4 with PP2Ac and S6K, an important target of the mTOR kinase, we performed co-immunoprecipitations with α4-V5 and MID1-FLAG overexpressing HeLa cells. Both, PP2Ac and S6K clearly co-precipitated with α4 and MID1 ( Supplementary Fig. S12 ). The interference between MID1, PP2A, mTOR and S6K made us ask the question if the effects of the MID1 protein on the translation efficiency of mRNAs with expanded CAG repeats are mediated by PP2A and mTOR activities. MID1 is a negative regulator of PP2Ac levels and activity. If the effect of the MID1 knockdown on the translation efficiency of the HTT mRNA with expanded CAG repeats was mediated by the influence of MID1 on PP2A activity, inhibition of PP2A—for example, by treatment with its inhibitor OA—should be able to rescue the seen effect. For an easier handling of cells and treatments in the luciferase assay we established a HeLa cell line that stably expresses the firefly luciferase gene carrying 51 CAG repeats in its 3′-UTR. PP2A dependency of the MID1 knockdown effect was analysed in a blocking experiment where these cells were transfected either with a non-silencing or with a MID1-specific siRNA oligonucleotide. In addition, cells were either mock treated or treated with OA, an inhibitor of PP2A. Results clearly show that the effect of MID1 knockdown on the synthesis of luciferase with 51 CAG repeats in its 3′-UTR can be completely blocked by OA treatment ( Fig. 6a ). 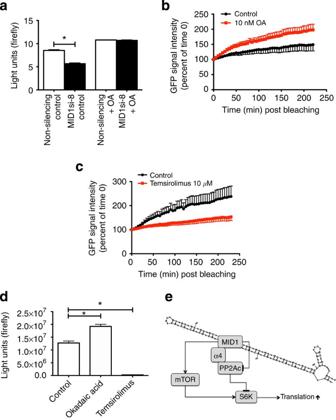Figure 6: Translation of mRNAs with expanded CAG repeats is PP2A and mTOR dependent. (a) Luciferase assay of a cell line stably expressing firefly luciferase carrying 51 CAG repeats in its 3′-UTR after transfection either with non-silencing control or MID1-specific siRNA oligonucleotides with or without okadaic acid (OA, 10 nM, 12 hours) treatment is shown. Samples were measured in triplicates. Mean values±s.d. are shown (P<0.05). (b) FRAP-based assay showing translation rates of the GFP-HTT-exon1 Q49 construct in HeLa cells treated with (n=35) or without OA (n=22). Data are presented as mean values±s.e.m. Curves showing signal recovery over time (P<0.0001) are depicted. (c) FRAP-based assay as inbshowing cells that were treated with (n=38) or without temsirolimus (n=29) (P<0.0001). Data are presented as mean values±s.e.m. (d) Luciferase assay of cells stably expressing firefly luciferase with 51 CAG repeats in its 3′-UTR. Cells were treated with or without either OA or temsirolimus. Samples were measured in triplicates. Mean values±s.d. are shown (P<0.05). (e) Model: HTT mRNA with expanded CAG repeats recruits a protein complex containing MID1, α4, PP2Ac and S6K. S6K induces protein translation and gets activated upon phosphorylation by mTOR. PP2A–as the mTOR opposing phosphatase–inactivates S6K by dephosphorylation. MID1 mediates binding of the protein complex to the CAG repeat mRNA and acts as a negative regulator of PP2A. MID1 also regulates mTOR activity: in the absence of MID1 PP2Ac binds to its subunits A and Bα (instead of binding MID1 and α4) and then inhibits binding of mTOR to its interacting proteins for example, raptor, which leads to inhibition of mTOR in this protein complex (called TORC1)19. Therefore, increased binding of MID1 and S6K to HTT mRNA with elongated CAG repeats leads to an increased protein translation. Figure 6: Translation of mRNAs with expanded CAG repeats is PP2A and mTOR dependent. ( a ) Luciferase assay of a cell line stably expressing firefly luciferase carrying 51 CAG repeats in its 3′-UTR after transfection either with non-silencing control or MID1-specific siRNA oligonucleotides with or without okadaic acid (OA, 10 nM, 12 hours) treatment is shown. Samples were measured in triplicates. Mean values±s.d. are shown ( P <0.05). ( b ) FRAP-based assay showing translation rates of the GFP-HTT-exon1 Q49 construct in HeLa cells treated with ( n =35) or without OA ( n =22). Data are presented as mean values±s.e.m. Curves showing signal recovery over time (P<0.0001) are depicted. ( c ) FRAP-based assay as in b showing cells that were treated with ( n =38) or without temsirolimus ( n =29) ( P <0.0001). Data are presented as mean values±s.e.m. ( d ) Luciferase assay of cells stably expressing firefly luciferase with 51 CAG repeats in its 3′-UTR. Cells were treated with or without either OA or temsirolimus. Samples were measured in triplicates. Mean values±s.d. are shown ( P <0.05). ( e ) Model: HTT mRNA with expanded CAG repeats recruits a protein complex containing MID1, α4, PP2Ac and S6K. S6K induces protein translation and gets activated upon phosphorylation by mTOR. PP2A–as the mTOR opposing phosphatase–inactivates S6K by dephosphorylation. MID1 mediates binding of the protein complex to the CAG repeat mRNA and acts as a negative regulator of PP2A. MID1 also regulates mTOR activity: in the absence of MID1 PP2Ac binds to its subunits A and Bα (instead of binding MID1 and α4) and then inhibits binding of mTOR to its interacting proteins for example, raptor, which leads to inhibition of mTOR in this protein complex (called TORC1) [19] . Therefore, increased binding of MID1 and S6K to HTT mRNA with elongated CAG repeats leads to an increased protein translation. Full size image PP2A is a negative regulator of protein translation and opposes mTOR kinase activity on the translation regulators S6K and 4E-BP1. Therefore, we asked if the translation of mRNAs with expanded CAG repeats is mTOR dependent. We performed the FRAP-based assay described above in the presence of either the mTOR inhibitor temsirolimus or the PP2A inhibitor OA. While OA significantly increased fluorescence recovery of HTT-exon1-GFP Q49 ( Fig. 6b , Supplementary Movie 4 , Supplementary Fig. S9 ), temsirolimus decreased the fluorescence recovery clearly ( Fig. 6c , Supplementary Movie 5 ). By contrast, OA treatment led to an only small increase of fluorescence recovery of HTT-exon1-GFP Q17 and temsirolimus had no effect on the fluorescence recovery of this construct ( Supplementary Fig. S13 ). The small OA effect can probably be explained by a residual MID1-binding ability of RNA with shorter CAG repeats, which we have seen in the RNA pull-down assays ( Fig. 1 ). In confirmation of the FRAP experiments, the cell line expressing firefly luciferase with 51 CAG repeats was treated with OA and temsirolimus. While OA stimulated luciferase production, temsirolimus almost entirely inhibited it ( Fig. 6d ). Together, these results demonstrate that the protein translation from mRNAs with expanded CAG repeats is an mTOR and PP2A-dependent mechanism. All these data indicate that the influence of the MID1-complex on the translation of HTT-exon 1 protein primarily affects mRNAs with CAG repeat expansions, but not with physiological repeat sizes and it involves PP2A/mTOR activity–probably via regulation of the translation regulator S6K. Expansion of CAG repeats is a common pathogenic mechanism in diseases like HD. Here we report a novel mechanism that regulates the translation of mRNAs with CAG repeat expansions. It involves MID1, PP2A and the PP2A/mTOR target S6K. Our data show that: (i) MID1, PP2Ac and S6K bind to CAG repeat stretches of the HTT mRNA in a repeat length dependent manner, (ii) protein synthesis increases with the size of the CAG repeat, (iii) knockdown of MID1 results in a significant reduction of protein produced from mRNAs containing elongated CAG repeats, an effect that can be blocked by PP2A inhibitors and (iv) treatment with PP2A and mTOR inhibitors has opposing effects on the translation efficiency of mRNAs carrying expanded CAG repeats. Until recently, solely the accumulation of polyQ-protein was believed to cause toxicity in polyQ expansion diseases like HD. Recent studies have shown that RNA–protein interactions of mutant poly-CAG RNAs might also contribute to toxicity: CAG repeat RNAs bind to and co-localize with the muscleblind (MBNL1) protein [12] . Originally MBNL1 had been found to bind to CUG or CCUG repeat mRNA-hairpin structures in patients with myotonic dystrophy (MD). In MD patients the sequestration of MBNL1 and other splicing factors by the mutant mRNAs leads to misregulated splicing, which is believed to be the underlying pathogenic mechanism in MD [34] , [35] , [36] . Similarly MBNL1 has been shown to bind CAG repeats [37] , [38] leading to dysregulated alternative splicing of target mRNAs in CAG repeat expansion disorders [39] . Furthermore, in a Drosophila model of Machado-Joseph disease, another CAG repeat expansion disorder, the MBNL1 protein enhanced CAG repeat RNA toxicity [8] , [34] , [35] , [36] , [37] , [38] . Thus, binding and sequestration of MBNL1 might be one possible mechanism contributing to RNA toxicity in CAG repeat expansion disorders (reviewed in Krzyzosiak et al. [40] ). Here we show that expanded CAG repeat stretches in the HTT mRNA bind to the MID1 protein complex and that this protein complex controls this mRNAs' translation. Elongated CAG repeats in HD patients, therefore, probably induce translation of pathological protein in a gain-of-function like manner by recruiting the MID1 protein complex. Remarkably, siRNA mediated interruption of the MID1–protein complex particularly influenced translation of mRNAs with longer–for example, pathological–CAG repeats and had no effect on mRNAs with normal repeat lengths. This indicates that by interfering with the MID1 protein complex it is possible to specifically influence protein translation from mRNAs carrying pathological sizes of repeats. These data make the MID1-complex a novel and very promising drug target for the development of a therapy for CAG repeat expansion disorders like HD aiming at the systematic reduction of pathological protein. HD is caused by the expansion of a CAG repeat, which translates into an expanded polyQ tract. The expanded polyQ stretch leads to an increased cleavage of mutant HTT by caspases and calpains, and results in an accumulation of toxic N-terminal HTT-fragments, which form aggregates in HD brains [41] , [42] , [43] , [44] , [45] . These fragments get degraded via the ubiquitin-proteasome pathway and by autophagy. Reduction of proteasomal degradation has been found in cells carrying CAG repeat expansions [46] , [47] , [48] , [49] and induction of both degradation pathways has been discussed as promising therapeutic strategies for CAG repeat expansion disorders including HD [50] , [51] , [52] , [53] . We show here that the MID1–PP2A complex controls the translation efficiencies of mRNAs that contain CAG repeat expansions. These findings suggest an RNA-based gain-of-function mechanism that leads to an overproduction of aberrant HTT protein in CAG repeat expansion carriers over time. The combination of both processes–a reduced clearance of mutant HTT protein plus an increase in translation of mutant HTT mRNA–could lead to a slow, over time accumulation of pathological protein in patients with HD. This would nicely explain (i) the slow accumulation of aggregates consisting of insoluble protein and (ii) the late onset of disease in CAG repeat expansion disorders. This hypothesis is further supported by data from Graham et al [54] . showing that in mice expressing varying levels of abnormal HTT protein increased protein levels account for a more severe phenotype, which is characterized by earlier onset, a more rapid progression and enhanced striatal volume loss. We also show that the translation of mutant HTT mRNA depends on PP2A and mTOR activities. Our data suggest that induction of PP2A or inhibition of mTOR would result in a significant reduction of translation of mutant protein in HD patients and thereby would be able to reduce protein aggregation and perhaps delay the development of the disease phenotype. Interestingly, induction of autophagy, which has an important role in the clearance of aberrant protein in CAG repeat expansion disorders, has also been linked to mTOR inhibition [52] . mTOR inhibitors, therefore, have significant potential in therapies of CAG repeat expansion disorders because they combine a reduction of the synthesis of aberrant protein with an increase of its degradation. Based on our observations we have developed a hypothetical working model: HTT mRNAs with pathologically expanded CAG repeats bind to the MID1 protein. MID1 recruits PP2Ac and the translation regulator S6K to these mRNAs. MID1 is a negative regulator of PP2Ac, thereby stimulating mTOR activity, the phosphorylation of S6K, and protein translation [19] . This then would lead to an overproduction of aberrant protein coded by the mRNA and its expanded CAG repeat stretch ( Fig. 6e ). RNA-structure prediction Structure predictions of bp 146–415 of the HTT-sequence NM_002111 with variable CAG repeat lengths were carried out using mfold (version 3.2) [55] , [56] . RNA pull-down HTT–CAG-repeat-motifs were PCR amplified, treated with proteinase K and purified by phenol–chloroform extraction. In vitro transcriptions were performed using the RiboMAX Large-scale RNA production system-T7 (Promega). The resulting biotinylated RNAs were purified by phenol–chloroform extraction. After preincubation of RNA with HeLa-protein extracts RNA pull-down was performed using streptavidin-coated Dynabeads (M-280, Dynal Biotech). RNAse assisted chromatography RNAse assisted chromatography was performed as described elsewhere [27] . In brief, HTT–CAG-repeat-motifs were PCR amplified, treated with proteinase K and purified by phenol–chloroform extraction. In vitro transcriptions were performed using the RiboMAX Large-scale RNA production system-T7 (Promega). The resulting RNAs were purified by phenol–chloroform extraction. After incubation of RNA with HeLa-protein extracts RNA–protein complexes were washed, RNA-bound proteins were eluted using RNAse, and proteins were analysed on western blots. Transient transfections and western blot Autophagy positive and negative cells (Atg +/+ and Atg −/−, MEFs from mice deficient for Atg5) (kindly provided by Dr Noboru Mizushima [29] ) were transfected with pEGFP-C1 and HTT-500AA-Q17/49, resuspended in Magic-Mix, and western blotted on polyvinylidene difluoride membranes (Roche). For quantification of western blots each sample was analysed in triplicates, band intensities were measured using Imagequant5.2. Data shown represent mean±s.d. Statistical significances were evaluated using t -test (two-tailed, homoscedastic). Expression constructs Expression-vectors were transfected using Lipofectamine 2000 (Invitrogen). Expression-vector constructs are listed ( Supplementary Table S1 ). In vitro translation Luciferase with CAG-repeat-motifs in the 3′-UTR was PCR amplified and subjected to in vitro transcription using the mMESSAGE mMACHINE Kit (Ambion). In vitro transcribed RNA was phenol–chloroform purified and analysed by means of in vitro translation using the Flexi Rabbit Reticulocyte Lysate System (Promega). Luciferase reporter assays U373MG/HeLa cells co-transfected with reporter plasmids (pGL3-vectors) and renilla luciferase (pRL) or a stable cell line expressing HTT-exon1 CAG 51 in the 3′-UTR of firefly luciferase (HeLa, TRex-system, Invitrogen) were subjected to luciferase reporter assays. Reporter assays were carried out using the Dual-Luciferase Reporter 1000 Assay System (Promega). Samples were analysed in quadruplicates. Data shown represent mean±s.d. Statistical significances were evaluated using t -test (two-tailed, homoscedastic). Real-time PCR Total RNA was isolated using the RNeasy Mini Kit (Qiagen). cDNA was synthesized using the TaqMan reverse transcription reagents kit (Applied Biosystems) and real-time PCR was carried out using the SYBRGreen PCR master mix (Applied Biosystems). Samples were analysed in quadruplicates. Data shown represent mean±s.d. Statistical significances were evaluated using t -test (two-tailed, homoscedastic). Primers Primers are listed in Supplementary Table S2 . Antibodies Antibodies are listed in Supplementary Table S3 . Short interfering RNAs siRNAs were transfected using Oligofectamine (Invitrogen) or Polyfect (Qiagen). Sequences of siRNAs are listed in Supplementary Table S4 . Filter retardation assay HEKT-cells stably expressing HTT-exon1 with 83 CAG repeats [3] were transfected with siRNAs. Filter retardation assays were performed as described elsewhere [3] . Samples were analysed in quadruplicates. Data shown represent mean±s.d. Statistical significances were evaluated using t- test (two-tailed, homoscedastic). HD-mice Wild-type or HD knock-in mice carrying 111 CAG repeats in the endogenous HTT -gene (B6.129-Htt tm5Mem /J, Jackson’s Lab stock No.003598) were decapitated and brains were rapidly dissected in nitrogen. Protein extracts were dissolved in Magic-Mix (48% urea, 15 mM Tris-HCL pH 7.5, 8.7% glycerine, 1% SDS, 0,004% Bromophenol blue, 143 mM Mercaptoethanol), separated on 6% SDS gels and analysed on western blots. Bands on the western blots were analysed in triplicates and quantified using Aida Image Analyser Software v.3.28. Data shown represent mean±s.d. Statistical significances were evaluated using t -test (two-tailed, homoscedastic). FRAP-based assays HeLa cells were transfected with constructs expressing HTT-exon1 fused to GFP. Twelve to twenty hours after transfection cells were analysed using a Zeiss LSM710NLO and a Zeiss LSM700 with a X20 objective. The GFP-signal of individual cells was bleached with a 488 argon laser of high intensity. Fluorescence signal was imaged over 4 h using reduced laser power to minimize photobleaching. Fluorescence signal was measured as the sum of the pixel over the cell area in each picture. The resulting total cell fluorescence was normalized for the whole time series to the second frame after bleaching, which was set to 100%. Bleaching experiments were performed on 14–38 cells for each experimental condition. Finally, mean values and s.e. values were calculated from normalized fluorescence recovery curves of single cells. To estimate statistical differences between different experimental conditions, normalized recovery curves of single cells were integrated over time (0–220 min) and rank-sum test was applied to distributions of resulting ‘area under the curve’ values. Co-immunoprecipitation For co-immunoprecipitation experiments, HeLa cells were transfected with MID1-FLAG and α4-V5. Forty-eight hours after transfection cells were lysed by sonication in IP-buffer (50 mM Tris pH 7.5, 2.5 mM MgCl 2 , 100 mM NaCl, 1 mM dithiothreitol, complete (protease inhibitor cocktail; Roche)) either with or without addition of RNAse (NEB). Immunoprecipitation was carried out using FLAG- or V5-specific antibodies or unspecific mouse IgG as negative controls in combination with protein A-/ or G-agarose (Roche) following the manufacturer’s instructions and immunoprecipitates were analysed on western blots. Statistical analysis Statistical analyses were performed using GraphPad Prism 5 software. Student’s t -test was used for two-group comparisons. For multiple comparisons data were analysed by one-way analysis of variance with post hoc Dunnett’s or Bonferonni test, as appropriate. For FRAP based assays, rank-sum test was applied to distributions of resulting ‘area under the curve’ values. How to cite this article: Krauß, S. et al. Translation of HTT mRNA with expanded CAG repeats is regulated by the MID1–PP2A protein complex. Nat. Commun. 4:1511 doi: 10.1038/ncomms2514 (2013).